Proliferation of neutral modes in fractional quantum Hall states The fractional quantum Hall effect is a canonical example of topological phases. While electric currents flow downstream in edge modes, neutral edge modes, observed only in hole-conjugate states and in ν =5/2, flow upstream. It is believed that the latter transport results from multiple counter-propagating channels—mixed by disorder that is accompanied by Coulomb interaction. Here we report on sensitive shot noise measurements that reveal unexpected presence of neutral modes in non-hole-conjugate fractional states; however, not in the integer states. Furthermore, the incompressible bulk is also found to allow energy transport. While density reconstructions along the edge may account for the energy carrying edge modes, the origin of the bulk energy modes is unidentified. The proliferation of neutral modes changes drastically the accepted transport picture of the fractional quantum Hall effects. Their apparent ubiquitous presence may explain the lack of interference of fractional quasiparticles—preventing observation of fractional statistics. Charge propagation in the quantum Hall effect regime takes place near the edge of the two-dimensional electron gas (2DEG) in the form of downstream chiral edge modes (with chirality determined by the direction of the magnetic field); while the bulk is incompressible (gapped) and thus does not contribute to the transport [1] , [2] , [3] , [4] . In the integer regime, with ν the integer filling factor (being the ratio between the number of electrons to the number of flux quanta, h / e ), charged excitations are electrons while in the fractional regime they are fractionally charged quasiparticles. However, as was predicted in the 1990s [5] , [6] , this picture is, in general, too simple. For, the so called, hole-conjugate states of the fractional quantum Hall effect (FQHE) regime, edge reconstruction of the electron density is expected to take place at the physical edge of the 2DEG; with counter-propagating edge currents. Since such edge currents were never observed, random tunnelling between these edge channels (owing to disorder), accompanied by Coulomb interaction, had been proposed to reorganize the multiple channels, leading to a downstream charge mode and upstream (counter propagating to the charge mode) neutral edge mode(s) [7] , [8] —as was indeed recently detected in hole-conjugate FQHE states [9] , [10] , [11] , [12] , [13] . Following a significant effort to develop a sensitive heat sensor in a thinly polished substrate [14] , our group detected the presence of neutral modes in ν =2/3, 3/5, 5/3, 8/3 and 5/2 via measuring noise, with zero net current, resulting from impinging the modes upstream on a partly pinched quantum point contact (QPC) constriction, or, alternatively, by on a non-ideal ohmic contact [9] , [10] , [11] . The measured noise may result from the fragmentation of the neutral quasiparticles (it is instructive to look at them as electric dipoles) by a partitioning barrier [9] , or, alternatively, owing to local Joule heating of the barrier [11] . Support to the latter mechanism was also provided by observing thermal broadening of conductance peaks [12] , where a nucleation of ν =2/3 state at the edge for the ν =1 bulk was observed at B =8.3T (not at B =6.2T), and the generation of net thermoelectric current at ν =2/3 (ref. 13 )—both in quantum dots. Though one can find predictions for edge reconstructions in particle-like fractional states [15] , [16] , [17] , [18] , [19] , [20] , the existence of upstream neutral modes in these fillings was not expected. Here we report on findings of upstream neutral edge modes, again via sensitive noise measurements, in particle-like fractional states. Moreover, and even more surprisingly, energy flow through the bulk was also found in all the tested fractional states. Note, that similar bulk heat transports in ν =1 (ref. 12 ) and in ν =4/3 (ref. 21 ) were recently reported. The presence of the excited neutral modes in the FQHEs, whether edge or bulk, may serve as possible decoherers (full or partial) of fractional quasiparticles in relation to experimental observations: high visibilities in the integer quantized Hall effects [22] and vanishing coherence in the FQHEs. Measurement set-up The employed samples were fabricated in several types of GaAs/AlGaAs heterostructures and each embeds a 2DEG (see Fig. 1 and Supplementary Fig. 1 for more details). The neutral modes, carrying energy, can be excited by two possible sources (see Fig. 1 and Supplementary Fig. 1 ), namely, a partly pinched QPC, which partitions downstream current I C arriving from S C (ref. 11 ) and the hot spot at the upstream side of a biased ohmic contact S N (ref. 9 ) fed by current I N . In the following experiments, neutral modes were converted to downstream current fluctuations, i 2 , with zero net current, in standard ohmic contacts. Voltage fluctuations, i 2 / v 2 G 0 2 (independent of the QPC transmission and G 0 = e 2 / h ), were amplified by a cryogenic preamplifier placed along the downstream edge at A CE , along the upstream edge at A NE or connected to the bulk at A NB . The presence of neutral modes was verified by measuring shot noise in two configurations ( Fig. 1 ): one is to partition I C by a QPC and measuring the resultant upstream noise at A NE and the bulk noise at A NB —named C→N, and the other configuration is to measure the noise at A CE in the presence of a neutral mode arriving upstream from S N —named C+N→C. The latter measurements allowed measuring the charge of the partitioned quasiparticles and their temperature in the presence of the impinged neutral current I N . It is worth reminding the reader of the ‘standard’ expression of excess noise (shot noise above the thermal contribution), owing to a stochastic partitioning (transmission t ) of a noiseless beam of charge e * quasiparticles, S i =2 e*It (1− t )(coth x − x −1 ) with x = e*I /2 k B ΘG 0 , where S i is the ‘zero frequency’ noise spectral density, k B the Boltzmann constant, e* the effective charge and I the impinged current [23] . We calibrated the differential transmission probability t by sourcing variable voltage DC+AC (0.5μ V RMS at 800 kHz) and measuring the AC voltage at contact A CE (more details are in Methods). 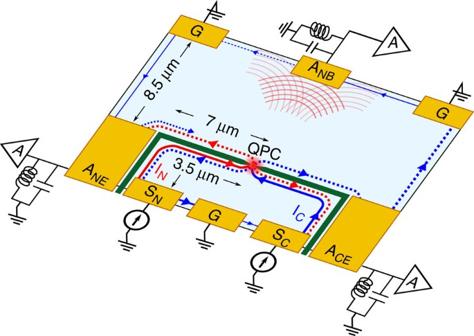Figure 1: Schematics of the experiment. The main device was fabricated in a GaAs/AlGaAs heterostructure with 2DEG embedded 130 nm below the surface whose density is 1.0 × 1011cm−2and the dark mobility is 5.1 × 106cm2V−1s−1at 4.2 K (seeSupplementary Fig. 1). The light-blue coloured region is the mesa embedding the 2DEG. The yellow pads are standard NiAuGe ohmic contacts, grounds (G), amplifiers (ACE, ANE& ANB), and sources, SCand SN, driving charge currentIC(blue thick arrows) and neutral currentIN(red thick arrow). The grounded contacts were tied directly to the cold finger of the dilution refrigerator. Heating the mixing chamber raised the temperature of the electrons. The QPC (green lines) was formed by negatively biased split-gates (10 nm Ti/30 nm Au) with a 660 nm wide opening, controlling the transmission probabilityt. The distance between SNand the QPC was 3.5 μm. Each amplifier contact was followed by a resonant circuit (peaking ~\n800 kHz) and a cryogenic voltage amplifier. ANEsits at 7 μm along the edge upstream from the QPC, measuring the upstream neutral edge mode solely. ANBis located at 8.5 μm over the mesa from the QPC, measuring the bulk mode solely. ACEwas to measure the noise in the downstream charge mode. Thin arrows are unbiased channels. We employed two configurations: first C→N, driving onlyIC, partitioned at the QPC and exciting the neutral modes if they were to exist, and detecting their presence by measuring the noise at ANEand ANBsimultaneously and second C+N→C, driving bothICandINand measuring the noise at ACE. The presence of the neutral modes can modify the effective charge and temperature of tunnelling quasiparticles. Figure 1: Schematics of the experiment. The main device was fabricated in a GaAs/AlGaAs heterostructure with 2DEG embedded 130 nm below the surface whose density is 1.0 × 10 11 cm −2 and the dark mobility is 5.1 × 10 6 cm 2 V −1 s −1 at 4.2 K (see Supplementary Fig. 1 ). The light-blue coloured region is the mesa embedding the 2DEG. The yellow pads are standard NiAuGe ohmic contacts, grounds (G), amplifiers (A CE , A NE & A NB ), and sources, S C and S N , driving charge current I C (blue thick arrows) and neutral current I N (red thick arrow). The grounded contacts were tied directly to the cold finger of the dilution refrigerator. Heating the mixing chamber raised the temperature of the electrons. The QPC (green lines) was formed by negatively biased split-gates (10 nm Ti/30 nm Au) with a 660 nm wide opening, controlling the transmission probability t . The distance between S N and the QPC was 3.5 μm. Each amplifier contact was followed by a resonant circuit (peaking ~\n800 kHz) and a cryogenic voltage amplifier. A NE sits at 7 μm along the edge upstream from the QPC, measuring the upstream neutral edge mode solely. A NB is located at 8.5 μm over the mesa from the QPC, measuring the bulk mode solely. A CE was to measure the noise in the downstream charge mode. Thin arrows are unbiased channels. We employed two configurations: first C→N, driving only I C , partitioned at the QPC and exciting the neutral modes if they were to exist, and detecting their presence by measuring the noise at A NE and A NB simultaneously and second C+N→C, driving both I C and I N and measuring the noise at A CE . The presence of the neutral modes can modify the effective charge and temperature of tunnelling quasiparticles. Full size image C→N in ν =2/3 We start with ν =2/3, where the presence of upstream neutral modes had been already established [9] , [11] , [12] , [13] . We fabricated a device with short propagation distance of the neutral modes, 3.5 μm and 7 μm, to enhance the measured shot noise. At the centre of the ν =2/3 conductance plateau, B =6.7T, with the state spin-polarized, the neutral mode was measured in the C→N configuration, with −4 nA≤ I C ≤4 nA ( Fig. 1 ). Another configuration, named N→N, relied on exciting the neutral mode by the ‘hot spot’ at the upstream side of S N by driving current I N . The neutral mode was partly transmitted by the upstream QPC and generated currentless noise at A NE (see Supplementary Fig. 2 ). In all the measurements, only a negligible amount of net current (<0.5 pA, via the bulk) was detected at A NE and A NB ; assuring a negligible contribution to the noise (if carrying Poissonian noise (see also Fig. 6b ), one would expect S i =2 eI bulk ~\n3 × 10 −31 A 2 Hz −1 ). A monotonically increasing (currentless) excess noise with I C was measured upstream along the edge (at A NE ) and directly through the bulk (at A NB ); both exhibiting ~\n t (1− t ) dependence [11] (see Fig. 2a,b ). Apparently, the excess noise along the edge in A NE , exhibiting a slight negative curvature, is some ten times higher than that in A NB . Note that the integrity of the state is maintained by keeping the excitation voltage in S C (150 μV) substantially lower than the presumed energy gap of v =2/3 (~\n780 μeV) [24] . Figure 6: Additional test of neutral modes in a top-gated device. We also investigated the presence of the neutral modes with a density-tunable device but without any QPC in the C→N configuration. ( a ) The 2DEG was embedded within the green region and the yellow pads are ohmic contacts (a source S C and an amplifier A NE to measure the C→N noise and grounds G). Note that this configuration does not measure the edge contribution and the bulk contribution separately. 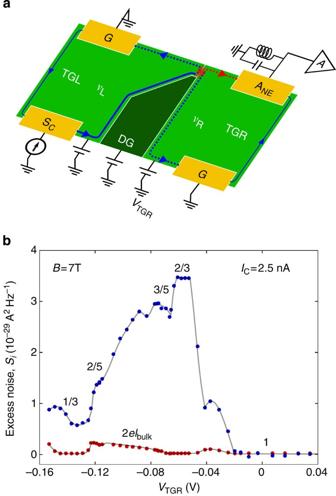Figure 6: Additional test of neutral modes in a top-gated device. We also investigated the presence of the neutral modes with a density-tunable device but without any QPC in the C→N configuration. (a) The 2DEG was embedded within the green region and the yellow pads are ohmic contacts (a source SCand an amplifier ANEto measure the C→N noise and grounds G). Note that this configuration does not measure the edge contribution and the bulk contribution separately. The blue (red) arrows depict the charge (neutral) current. Top gates, coloured in light green, for the left (TGL) and right halves (TGR) of the mesa tuned the local filling factorsνLandνR, respectively. We variedνRby the gate voltageVTGRon TGR and adjustedνLto be at 1 throughout the experiment. The defining gate (DG) in dark-green always fully depleted the 2DEG underneath. The density of 2DEG atVTGR=0 V was 1.3 × 1011cm−2. The interface of the left and right top gates was 3 μm and the path length between the interface and the amplifier contact was 8 μm. (b) AtB=7 T, drivingIC=2.5 nA, the C→N noise as a function ofVTGRwas measured (blue dots) simultaneously with the bulk currentIbulk, measured separately, (the Poissonian noise 2eIbulkin red dots). The filing fractions (νR=1/3, 2/5, 3/5, 2/3 and 1) were specified along the plot. The noise stayed finite at all the fillings except forνR=1 and but gradually went down towardsνR=1/3, which is compatible with the observations shown above. Particularly, it is notable that, upon approachingνR=1/3 afterνR=2/5, the bulk current vanished while the noise increased. The blue (red) arrows depict the charge (neutral) current. Top gates, coloured in light green, for the left (TGL) and right halves (TGR) of the mesa tuned the local filling factors ν L and ν R , respectively. We varied ν R by the gate voltage V TGR on TGR and adjusted ν L to be at 1 throughout the experiment. The defining gate (DG) in dark-green always fully depleted the 2DEG underneath. The density of 2DEG at V TGR =0 V was 1.3 × 10 11 cm −2 . The interface of the left and right top gates was 3 μm and the path length between the interface and the amplifier contact was 8 μm. ( b ) At B =7 T, driving I C =2.5 nA, the C→N noise as a function of V TGR was measured (blue dots) simultaneously with the bulk current I bulk , measured separately, (the Poissonian noise 2 eI bulk in red dots). The filing fractions ( ν R =1/3, 2/5, 3/5, 2/3 and 1) were specified along the plot. The noise stayed finite at all the fillings except for ν R =1 and but gradually went down towards ν R =1/3, which is compatible with the observations shown above. 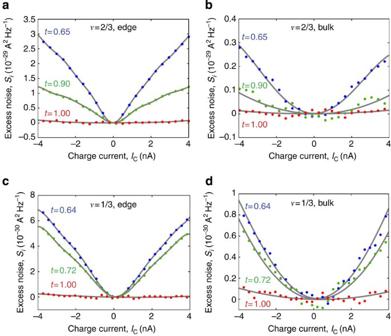Particularly, it is notable that, upon approaching ν R =1/3 after ν R =2/5, the bulk current vanished while the noise increased. Figure 2: C→N noise atν=2/3 and 1/3 for several QPC transmissions. The configuration C→N allows us to detect the neutral modes in the upstream edge and over the bulk separately. (a) Inν=2/3, the C→N noise at ANEfor −4 nA≤IC≤4 nA with transmissionst=0.65, 0.90 and 1.00. As|IC| increases, the noise also increases monotonically. The magnitude of the noise approximately goes ast(1−t). (b) Inν=2/3, the C→N noise at ANBmeasured simultaneously with ANE. The magnitude of the noise in ANBis about 10 times smaller than that in ANE. (c) Inν=1/3, the C→N noise at ANEfor −4 nA≤IC≤4 nA with transmissionst=0.64, 0.72 and 1.00. The noise again increases monotonically with|IC|. The magnitude of the noise follows nearlyt(1−t). (d) Inν=1/3, the C→N noise at ANBmeasured simultaneously with ANE. The magnitude of the noise in ANBis about seven times weaker than that in ANE. Full size image Figure 2: C→N noise at ν =2/3 and 1/3 for several QPC transmissions. The configuration C→N allows us to detect the neutral modes in the upstream edge and over the bulk separately. ( a ) In ν =2/3, the C→N noise at A NE for −4 nA≤ I C ≤4 nA with transmissions t =0.65, 0.90 and 1.00. As |I C | increases, the noise also increases monotonically. The magnitude of the noise approximately goes as t (1− t ). ( b ) In ν =2/3, the C→N noise at A NB measured simultaneously with A NE . The magnitude of the noise in A NB is about 10 times smaller than that in A NE . ( c ) In ν =1/3, the C→N noise at A NE for −4 nA≤ I C ≤4 nA with transmissions t =0.64, 0.72 and 1.00. The noise again increases monotonically with |I C |. The magnitude of the noise follows nearly t (1− t ). ( d ) In ν =1/3, the C→N noise at A NB measured simultaneously with A NE . The magnitude of the noise in A NB is about seven times weaker than that in A NE . Full size image C+N→C in ν =2/3 In the C+N→C configuration at filling v =2/3, we measured the noise at A CE in the range −4 nA≤ I C ≤4 nA and 0 nA≤ I N ≤4 nA ( Fig. 3 ). Two contributions to the downstream excess noise at A CE were measured ( Fig. 3a ): one owing to partitioning of I C in the presence of I N , and the other owing to fragmentations of the neutral mode arriving from S N (or excess heating). Assuming these are uncorrelated contributions, we can easily extract the temperature and charge of the partitioned quasiparticles (note, that detailed mechanism of neutral-charge interaction in the QPC is not known) [9] , [10] , [11] . At I N =0, with increasing I C the excess noise monotonically increases (above expression), with the partitioned quasiparticle charge e *~\n2 e /3 at temperature T =25 mK ( Fig. 3b ). As I N increased from 0–4 nA, the contribution of the neutral mode to the noise increased, and the partitioned quasiparticle charge gradually decreased from e *~\n2 e /3 to e *~\n0.4 e . Similarly, the temperature of the partitioned quasiparticles increased to ~\n140 mK at I N =4 nA, as shown in Fig. 3c ; agreeing qualitatively with previous measurements [9] , [25] . 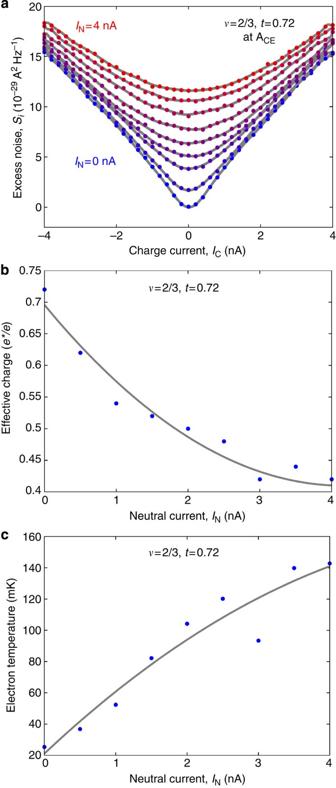We note that such temperature increase barely influenced the transmission t of the QPC as observed in the preceding study [9] . Figure 3: C+N→C noise atν=2/3. The influence of the currentINon partitioning the charge currentICalso provides indications of the presence of the neutral modes. (a) The C+N→C noise at ACEfor −4 nA≤IC≤4 nA witht=0.72 was measured in the presence of 0 nA≤IN≤4 nA in steps of 0.5 nA. While the traces are merging at highICregion, one can clearly see an increase in the cut atIC=0 nA, which is consistent with the C→N measurement and shows the N→C process is also present. Note that the transmission as a function ofICwas barely affected by the presence ofIN. (b) The extracted effective charge as a function ofINshows the suppression of the effective charge, approximately from 2e/3 down toe/3, as reported before. (c) The fitted temperature as a function ofINshows the rise of the electron temperature, from about 20 mK up to 140 mK, with increasingIN. Figure 3: C+N→C noise at ν =2/3. The influence of the current I N on partitioning the charge current I C also provides indications of the presence of the neutral modes. ( a ) The C+N→C noise at A CE for −4 nA≤ I C ≤4 nA with t =0.72 was measured in the presence of 0 nA≤ I N ≤4 nA in steps of 0.5 nA. While the traces are merging at high I C region, one can clearly see an increase in the cut at I C =0 nA, which is consistent with the C→N measurement and shows the N→C process is also present. Note that the transmission as a function of I C was barely affected by the presence of I N . ( b ) The extracted effective charge as a function of I N shows the suppression of the effective charge, approximately from 2 e /3 down to e /3, as reported before. ( c ) The fitted temperature as a function of I N shows the rise of the electron temperature, from about 20 mK up to 140 mK, with increasing I N . Full size image C→N in ν =1/3 We move now to ν =1/3, where neutral modes were not observed before and, while not forbidden theoretically, their presence was not expected. Employing first the C → N configuration, with the magnetic field tuned to the centre of the conductance plateau, B =13.5T. As shown in Fig. 2c,d , excess upstream noise was observed, accompanied also by noise in A NB . Though considerably weaker than in ν =2/3, the excess noise was easily detected (owing to the shorter propagation length compared with that in ref. 9 and the extremely ‘quiet’ preamplifiers), exhibiting also ~\n t (1− t ) dependence; with the noise along the edge some eight time stronger than that through the bulk. As in the v =2/3 case, the excitation voltage is maintained much smaller than the gap energy [24] . C+N→C in ν =1/3 Measurements at the C+N→C configuration followed at ν =1/3 ( Fig. 4 ). The excess noise followed the familiar dependence on current; however, the partitioned quasiparticle charge varied with the bias (even though t was constant). Concentrating on the small bias regime ( I C <2 nA), the partitioned quasiparticle charge (at I N =0) was e *~\n0.78 e ( Fig. 4b ). This is not surprising, as quasiparticle bunching is often found when t is not nearly unity [26] . As I N increased, the quasiparticle charge decreased to e *=0.56 e , accompanied by temperature increase of the partitioned quasiparticles to ~\n85 mK ( Fig. 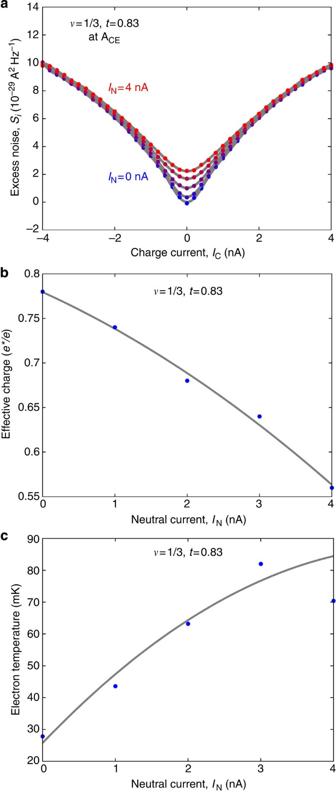4c ). Figure 4: C+N→C noise atν=1/3. Another verification of the neutral mode inν=1/3 in the C+N→C configuration. (a) The C+N→C noise at ACEfor −4 nA≤IC≤4 nA witht=0.83 was tested with 0 nA≤IN≤4 nA in steps of 1 nA. A distinct increase in the low |IC| region (≤2 nA) showed up, again being consistent with the C→N measurement and witnessing the N→C process. Note thatINhad negligible effect on the transmission as a function ofIC. (b) The effective charge as a function ofINdecayed approximately from 0.8edown to 0.5e, relaxing the quasiparticles bunching, similar to a previous study. (c) The electron temperature as a function ofINrose from about 25 mK up to 80 mK with increasingIN. Figure 4: C+N→C noise at ν =1/3. Another verification of the neutral mode in ν =1/3 in the C+N→C configuration. ( a ) The C+N→C noise at A CE for −4 nA≤ I C ≤4 nA with t =0.83 was tested with 0 nA≤ I N ≤4 nA in steps of 1 nA. A distinct increase in the low | I C | region (≤2 nA) showed up, again being consistent with the C→N measurement and witnessing the N→C process. Note that I N had negligible effect on the transmission as a function of I C . ( b ) The effective charge as a function of I N decayed approximately from 0.8 e down to 0.5 e , relaxing the quasiparticles bunching, similar to a previous study. ( c ) The electron temperature as a function of I N rose from about 25 mK up to 80 mK with increasing I N . Full size image C→N in other fillings Having established the presence of currentless neutral modes in ν =2/3 and also in the unexpected ν =1/3 states, we also tested other particle-like states, such as ν =2/5 and ν =4/3. In both cases, only the current carried by the inner channels (2/5–1/3, and 4/3–1) was partitioned by the QPC in the C→N configuration. The results are qualitatively similar to those in ν =1/3 states. (see Supplementary Fig. 3 for C→N configuration at ν =2/5). Though it cannot be fully discounted [12] , integer fillings ( ν =1 at B =4.4 T and 5.4 T) did not have any measurable noise in the C→N configuration; even with I C =4 nA and background noise level <5 × 10 −31 A 2 Hz −1 (see Supplementary Fig. 4 ). C→N at various temperatures Since spurious thermal effects may contribute to the excess noise, measurements in the C→N configuration were repeated at temperature T =50, 100 and 180 mK at ν =2/3 and ν =1/3. Strong reduction of the excess noise at A NE and A NB was observed ( Fig. 5 ). Such noise suppression indicates that the minute bulk current, which increased slightly with temperature (since R xx increased), does not contribute to the excess noise and that the decay of the excess noise with temperature conforms qualitatively with the expected shortening of the decay length with temperature [7] , [8] . Note that the bulk mode seems to decay much faster in comparison with the edge mode. 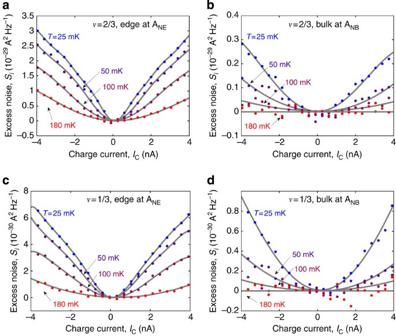Having both similar propagation lengths, it may suggest that the modes are of two different natures. Figure 5: C→N noise atν=2/3 and 1/3 at elevated temperatures. We repeated the measurement of the C→N noise at 50, 100 and 180 mK forν=2/3 and 1/3 at both amplifiers. In all the cases, the noise decayed with raising the temperature. The bulk noise weakened faster than the edge noise, indicating that the two noises were mediated by different modes. (a) Inν=2/3, the C→N noise measured at ANEfor −4 nA≤IC≤4 nA witht=0.65. (b) Inν=2/3, the C→N noise measured at ANBsimultaneously with ANE. (c) Inν=1/3, the C→N noise measured at ANEfor −4 nA≤IC≤4 nA with transmissionst=0.64. (d) Inν=1/3, the C→N noise measured at ANBsimultaneously with ANE. Figure 5: C→N noise at ν =2/3 and 1/3 at elevated temperatures. We repeated the measurement of the C→N noise at 50, 100 and 180 mK for ν =2/3 and 1/3 at both amplifiers. In all the cases, the noise decayed with raising the temperature. The bulk noise weakened faster than the edge noise, indicating that the two noises were mediated by different modes. ( a ) In ν =2/3, the C→N noise measured at A NE for −4 nA≤ I C ≤4 nA with t =0.65. ( b ) In ν =2/3, the C→N noise measured at A NB simultaneously with A NE . ( c ) In ν =1/3, the C→N noise measured at A NE for −4 nA≤ I C ≤4 nA with transmissions t =0.64. ( d ) In ν =1/3, the C→N noise measured at A NB simultaneously with A NE . Full size image C→N with density-tunable device To verify further the presence of upstream neutral modes in particle-like states, we employed a different geometry, which allowed continuous tuning of the filling fraction in the bulk via top gates; albeit not separating the bulk and edge contributions (see Fig. 6a ). We employed the C→N configuration ( I C =2.5 nA); however, instead of partitioning the edge channel with a QPC as above, it was partitioned at the interface between two filling factors: arriving from v L =1 region and partitioned into a variable v R <1 region—with an assumed ‘hot spot’ at the partitioned region (see Fig. 6a ). The length of the interface between top gate left (TGL) and top gate right (TGR) was 3 μm and the total path length to the amplifier contact was 8 μm. The upstream neutral mode was expected to propagate in the v R <1 region, with noise produced in ohmic contact A NE . In Fig. 6b we plotted the measured noise at B =7 T as a function of the gate voltage on the right top gate V TGR as well as the undesirable bulk current I bulk as its presumed Poissonian noise 2 eI bulk . Evidence of upstream noise is clear in all fractional fillings between v R =2/3 and v R =1/3. Note that while the bulk current goes up in the compressible regions, the noise goes down – as was described above. As before, the noise in the particle-like states is considerably smaller than in v R =2/3 with vanishing bulk current in both cases. Varying the density of the bulk and adjusting correspondingly the magnetic field, we also performed noise measurements at constant filling fractions, with the results shown in some details in the Supplementary Fig. 5 . The discovery of the proliferation of neutral modes changes the accepted view of current and energy transport by chiral edge channels and the bulk in the FQHE. Though only a few fractional states had been tested here it is highly likely that most fractional states, whether particle-like or hole-like, harbour a much more complex edge structures. Moreover, the bulk, despite of being incompressible, seems to be active energetically. Since the topological properties of the bulk dictate a conserved quantum thermal conductance for each state (for example, zero for v =2/3; one for v =1/3) [27] , it imposes fundamental differences between particle-like and hole-like states. Even for a sharp confinement potential (compared with magnetic length), the v =2/3 state must consist of two oppositely propagating channels while the v =1/3 is likely to possess a single downstream channel. Moreover, rather than having only two oppositely propagating edge channels in the v =2/3 state, for a shallow enough confining potential, an additional puddle of v =1/3 state can nucleate on the edge (thus adding a pair of counter-propagating 1/3 channels) [28] , [29] . In fact, our measurements were performed with ‘gate defined’ 2D structures (see Fig. 1 ), and thus, the electron density decreased gradually towards the edge—encouraging such edge reconstruction. Hence, such edge reconstruction might be eliminated in the latter, by sharpening the edge confinement potential, and thus affecting the presence and the nature of the neutral modes. How can one envision the likely edge reconstruction in v =1/3 state? Very much like the parameters that play a role in the v =2/3 state, a competition among the confinement potential, magnetic length and the Coulomb interaction, dictates the electron distribution near the edge [28] , [29] . The electron density should, at first, decrease monotonously towards the edge, leading to a downstream channel. Subsequently, two (at least) counter-propagating channels must emerge: one upstream owing to an increased electron density, and one downstream owing to the density dropping to zero at the depletion region near the edge. Yet, the net conductance must be G 0 /3; necessitating an upstream neutral mode. It is unlikely that the two added channels should be of v =1/3 character; since the original 1/3 channel and the added upstream one will easily localize owing to disorder [30] . Hence, the added two channels may be of lower filling, such as v =1/5, or, alternatively, a higher one, such as v =1. This type of reconstruction may depend on details and should be confirmed experimentally at each fractional filling. The presence of bulk modes may indicate bulk-edge coupling, even though some of the features and temperature dependence are different [12] , [21] . We are not aware of any prediction of such bulk energy transport, specifically in the fractional regime, which may account for our observation. The immeasurably small noise in A NB in the integer regime likely eliminates energy transport via crystal phonons emerging from the region of potential imbalance (ohmic contact or QPC). The proliferation of energy modes, especially those excited by partitioning of current in a QPC, may explain the difficulty in observing interference of fractional charges in interferometers that are based on charge partitioning. Drawing energy from the charged quasiparticles in the partitioning process, the modes may serve as sources of decoherence—preventing studying the statistics of fractionally charged quasiparticles. For the noise measurement, a voltage source with 1 GΩ resistor at its output fed the DC currents and the generated noise signals at amplifier contacts, filtered with an LC circuit tuned to ~\n800 kHz, were amplified first by a cooled, home-made, preamplifier with voltage gain 11 and subsequently by a room temperature amplifier (NF-220F5) with voltage gain 200. The amplified signal was measured by a spectrum analyzer with the bandwidth of 10 kHz. To monitor the net current reaching the amplifiers A NE and A NB , 5 μ V RMS at the resonant frequency on top of the DC currents was applied from the sources and measured at amplifiers with the bandwidth of 30 Hz. For the differential conductance measurement to characterize the QPC, we sent 0.5 μ V RMS at the resonant frequency along with DC currents and measured at A CE with the bandwidth of 30 Hz. See the Supplementary Fig. 1 for more details on the sample description. How to cite this article: Inoue, H. et al. Proliferation of neutral modes in fractional quantum Hall states. Nat. Commun. 5:4067 doi: 10.1038/ncomms5067 (2014).